Dynamic phosphorylation of HP1α regulates mitotic progression in human cells Heterochromatin protein 1α (HP1α), a key player in the establishment and maintenance of higher-order chromatin regulates key cellular processes, including metaphase chromatid cohesion and centromere organization. However, how HP1α controls these processes is not well understood. Here we demonstrate that post-translational modifications of HP1α dictate its mitotic functions. HP1α is constitutively phosphorylated within its amino terminus, whereas phosphorylation within the hinge domain occurs preferentially at G2/M phase of the cell cycle. The hinge-phosphorylated form of HP1α specifically localizes to kinetochores during early mitosis and this phosphorylation mediated by NDR1 kinase is required for mitotic progression and for Sgo1 binding to mitotic centromeres. Cells lacking NDR kinase show loss of mitosis-specific phosphorylation of HP1α leading to prometaphase arrest. Our results reveal that NDR kinase catalyses the hinge-specific phosphorylation of human HP1α during G2/M in vivo and this orchestrates accurate chromosome alignment and mitotic progression. Post-translational modifications of proteins regulate epigenetic control of gene expression. Modifications in histone and non-histone proteins dictate higher-order chromatin structure that in turn modulates gene silencing and chromosome segregation [1] , [2] . Heterochromatin is a specialized state of higher-order chromatin that typically represents gene poor, highly condensed and transcriptionally silent regions and is characterized by the presence of histone H3K9 trimethylation marks [3] , [4] . Heterochromatin protein 1 (HP1) is the key reader of this histone mark and is responsible for recruiting other effector molecules that together establish the heterochromatin domain [5] , [6] . HP1 consists of an amino-terminal chromodomain (CD) that recognizes and binds to methylated H3K9 (ref. 4 ), a carboxy-terminal chromoshadow domain (CSD) responsible for HP1 dimerization and protein–protein interaction [7] , [8] , [9] and a flexible hinge (H) region of variable length that separates the chromo and chromo shadow domains and is also thought to mediate chromatin binding [10] , [11] . The interactions of several histone and non-histone proteins with the isoforms of HP1 (α, β and γ) in mammalian cells have already been implicated in essential cellular process, including the establishment and maintenance of higher-order chromatin, metaphase chromatid cohesion and centromere architecture [5] , [12] , [13] . Post-translational modifications to all isoforms of HP1 at both CD and CSD modulate its interaction with other proteins or histone marks or regulate its function [14] , [15] , [16] . Protein phosphorylation is a key regulatory post-translational event that controls protein function and localization [17] . The interplay between protein kinases and their specific substrates dictate crucial cellular processes ranging from cell cycle progression to chromatin organization. HP1, originally identified from a silenced region of Drosophila polytene chromosome, is hyperphosphorylated by casein kinase II (CKII) [18] , [19] , [20] , [21] , [22] . In Drosophila , the hyperphosphorylation of HP1 is implicated with heterochromatin assembly [18] , whereas hypophosphorylated HP1 remains in a complex with a high mobility group (HMG)-like HP1/origin recognition complex -associated protein (HOAP) and origin recognition complex (ORC) [23] . Since the discovery of HP1 in Drosophila , orthologues have been identified in various species including fission yeast, chicken, mouse and human with remarkable evolutionary conservation [7] , [24] , [25] , [26] . Similarly, the phosphorylation of the fission yeast homologue of HP1, Swi6, regulates the binding of transcription regulators to chromatin and affects the transcriptional status at the heterochromatin [27] . Swi6 phosphorylation by CKII is required for gene silencing but not for chromosome segregation and sister chromatid cohesion, suggesting that independent mechanisms regulate each of these events [28] . Hsk1, another protein kinase, also interacts with Swi6 and is required for heterochromatic gene silencing, suggesting that multiple kinases may be involved in phosphorylating Swi6 (ref. 29 ). Mammalian HP1 is also highly phosphorylated and phosphorylation of HP1α at the N-terminal serine residues imparts stronger binding affinity to methylated H3K9 resulting in more robust chromatin association [14] , [30] , [31] . CKII phosphorylates HP1β at the chromo shadow domain following DNA damage that in contrast results in disruption of chromatin binding of HP1β [32] . Although in vitro data suggest that CKII can phosphorylate HP1α, there is no in vivo evidence that supports the role of CKII in HP1α phosphorylation. The elucidation of the biological function of phosphorylation of HP1α and the identification of an in vivo kinase that phosphorylates HP1α in mammals remain elusive. Nuclear Dbf2-related (NDR) kinases are highly conserved kinases that control vital cellular processes in various organisms, including mitotic exit, cytokinesis, cell growth, and proliferation and differentiation [33] . The NDR kinase orthologues have been shown to be required for the mitosis exit network in budding yeast and for septation initiation network in fission yeast [34] , [35] , [36] . Dbf2 orthologues in close association with upstream Ste-20-like kinases and Mps-one-binding (MOB) co-activators together constitute the Hippo pathway and coordinate key cellular processes like cell growth, proliferation and tumorigenesis [37] , [38] , [39] . In humans, NDR kinases have been shown to be required for G1/S transition, centrosome duplication and for mitotic chromosome alignment [40] . To date, the cell cycle protein p21 is the only known in vivo substrate identified for NDR kinase in human cells [40] . Recent work demonstrated that NDR1 kinase is required for accurate chromosome alignment [41] but the relevant substrates remain to be identified. In this study, we have identified that NDR kinase phosphorylates HP1α within its hinge domain predominantly during G2/M phase of the cell cycle. During early mitosis, hinge-phosphorylated HP1α localizes to kinetochores. Depletion of NDR kinase results in chromosomal alignment defects associated with defects in phosphorylation of HP1α at the hinge region and disruption of human Shugoshin (Sgo1) binding to centromeres. Our results demonstrate that NDR1 kinase-mediated phosphorylation of HP1α is required for accurate chromosome alignment and mitotic progression in mammalian cells. NDR kinase associates with HP1α In a screen to identify the substrates for NDR kinases, we have detected HP1α, a protein that regulates heterochromatin organization and cell cycle progression, as an NDR kinase-interacting protein. To verify the interaction between NDR kinase and HP1α, we co-transfected haemagglutinin (HA)-NDR1 and YFP-HP1α, followed by HA immunoprecipitations to demonstrate the interaction of NDR1 with HP1α ( Fig. 1a and Supplementary Fig. 1a ). Similarly, transient transfection of HA-HP1α and T7-NDR1 followed by immunoprecipitation using HA antibody confirmed the interaction of NDR1 and HP1α ( Fig. 1b and Supplementary Fig. 1b ). 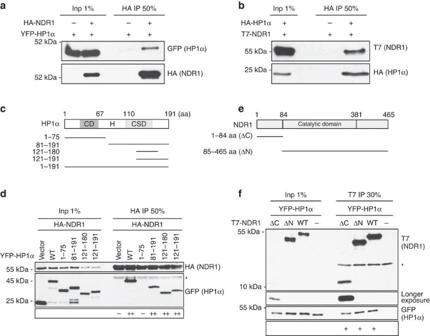Figure 1: NDR1 associates with HP1α. (a) Immunoprecipitation using HA antibody in cells expressing YFP-HP1α with (+) or without (−) HA-NDR1. Note the interaction between HA-NDR1 and YFP-HP1α (detected by GFP immunoblot). (b) Reciprocal immunoprecipitation using HA antibody in cells expressing T7-NDR1 with (+) or without (−) HA-HP1α. (c) Schematic representation of HP1α truncation mutants. (d) Immunoprecipitation using HA antibodies from cells expressing HA-NDR1 along with HP1α truncation mutants. Immunoblots using GFP antibody demonstrate robust interaction of NDR1 kinase with the mutants containing the CSD (121–180/191) or with CSD and hinge region (81–191) but not with the chromo domain (1–75 amino acids). YFP vector transfected with HA-NDR1 has been used as a control. Extent of interaction is depicted below the immunoblots. (e) Schematic representation of truncation mutants of NDR1 kinase spanning hydrophobic N-terminal as well as the central catalytic/kinase domain. (f) Immunoprecipitation using T7 antibody from cells expressing YFP-HP1α and various truncation mutants of T7-NDR1 (ΔC and ΔN). Note that HP1α interacts with both the N and C terminus of the NDR1 kinase. Extent of interaction is depicted below the immunoblots. Figure 1: NDR1 associates with HP1α. ( a ) Immunoprecipitation using HA antibody in cells expressing YFP-HP1α with (+) or without (−) HA-NDR1. Note the interaction between HA-NDR1 and YFP-HP1α (detected by GFP immunoblot). ( b ) Reciprocal immunoprecipitation using HA antibody in cells expressing T7-NDR1 with (+) or without (−) HA-HP1α. ( c ) Schematic representation of HP1α truncation mutants. ( d ) Immunoprecipitation using HA antibodies from cells expressing HA-NDR1 along with HP1α truncation mutants. Immunoblots using GFP antibody demonstrate robust interaction of NDR1 kinase with the mutants containing the CSD (121–180/191) or with CSD and hinge region (81–191) but not with the chromo domain (1–75 amino acids). YFP vector transfected with HA-NDR1 has been used as a control. Extent of interaction is depicted below the immunoblots. ( e ) Schematic representation of truncation mutants of NDR1 kinase spanning hydrophobic N-terminal as well as the central catalytic/kinase domain. ( f ) Immunoprecipitation using T7 antibody from cells expressing YFP-HP1α and various truncation mutants of T7-NDR1 (ΔC and ΔN). Note that HP1α interacts with both the N and C terminus of the NDR1 kinase. Extent of interaction is depicted below the immunoblots. Full size image To map the interacting domains between HP1α and NDR1, various truncation mutants of HP1α, 1–75 amino acids (spanning the chromo domain); 81–191 amino acids (hinge and CSD); 121–180 and 121–191 amino acids (CSD) were generated ( Fig. 1c ). Co-transfection of HA-NDR1 along with YFP vector or YFP-HP1α full length or truncation mutants, followed by immunoprecipitation using HA antibody revealed the association of NDR1 predominantly with the CSD of HP1α ( Fig. 1d ). This is further confirmed by the fact that a CSD mutant of HP1α that has lost its ability to bind PXVXL/I ligands (HP1α–W174A) failed to interact with NDR1 ( Supplementary Fig. 1b ). To identify the NDR1 domain that associates with HP1α, we generated NDR1 truncation mutants, 1–84 amino acids (spanning N-terminal regulatory sequence, ΔC) and 85–465 amino acids, (containing a C-terminal hydrophobic motif and the catalytic domain, ΔN; Fig. 1e ). Co-immunoprecipitation (Co-IP) of these mutants with HP1α demonstrated that multiple regions on NDR1 interacted with HP1α ( Fig. 1f ). To study the association of NDR kinases with HP1α at an in vivo locus, we used a cell line originally developed by Spector and colleagues [42] . The locus has several hundred copies of the lac operator repeats that can be easily visualized by the presence of a Cherry-lac repressor (LacI) [43] , [44] ( Fig. 2a,b ). We generated a triple fusion protein consisting of YFP-LacI-HP1α and examined whether the accumulation of HP1α at the site was sufficient to recruit NDR1 to that site. In addition to the tethered chromatin locus, a fraction of the YFP-LacI-HP1α was also present at heterochromatic regions within the nucleus that is apparent on overexposure ( Supplementary Fig. 1c ). CFP-NDR1 is predominantly a cytoplasmic protein with low amounts of it being detected in the nucleus. However, on tethering of HP1α, the CFP-NDR1 was present in the nuclear chromatin site in 18% of the cells ( Fig. 2b ). We also co-expressed CFP-NDR1-1-84aa (CFP-NDR1-ΔC, Fig. 2b ) or CFP-NDR1-85-465aa (CFP-NDR1-ΔN, Fig. 2b ) in YFP-LacI-HP1α-expressing cells. CFP-NDR1-85-465 (ΔN) was recruited to the chromatin locus in similar percentage of the cells (19%; Fig. 2b ). CFP-NDR1 expressing only the N terminus (1–84 amino acids), CFP-NDR1-ΔC, was predominantly localized in the nucleus, suggesting that the C terminus of this kinase contains a nuclear export signal. The nuclear enriched CFP-NDR1-ΔC accumulated at the YFP-LacI-HP1α-tethered locus in 37% of cells ( Fig. 2b ). Similar to the in vitro results, both ΔC- and ΔN-NDR1 mutants were found to associate with the HP1α-tethered chromatin locus. We observed a weak signal of NDR1 kinase at the CLTon locus ( Fig. 2b ) since the endogenous HP1α is known to localize to these sites [42] . However, the signal intensity of NDR1 when HP1α is tethered to the locus was much higher than when HP1α is not tethered. 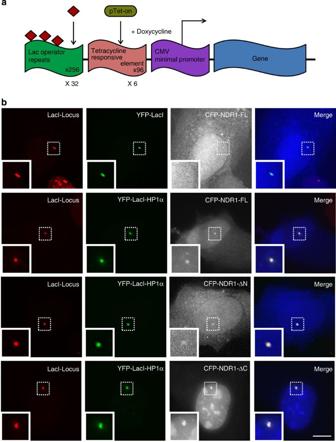Figure 2: Association of NDR1 with HP1α at anin vivoreporter heterochromatic locus. (a) Schematic representation of the U2OS 2-6-3 CLTon array that has been stably integrated in human cells (adapted and modified42,43,44). (b) The chromatin locus is visualized by Cherry-LacI staining. Cells were co-transfected with YFP-LacI and CFP-NDR-FL or with YFP-LacI-HP1α and CFP-NDR1 or its truncation mutants. YFP-LacI does not recruit CFP-NDR1 to the locus, whereas YFP-LacI-HP1α can efficiently recruit CFP-NDR1 to the chromatin locus. Cells co-transfected with YFP-LacI-HP1α and CFP-NDR1-ΔN or CFP-NDR1-ΔC shows accumulation at the HP1α containing locus. Scale bar, 10 μm. Figure 2: Association of NDR1 with HP1α at an in vivo reporter heterochromatic locus. ( a ) Schematic representation of the U2OS 2-6-3 CLTon array that has been stably integrated in human cells (adapted and modified [42] , [43] , [44] ). ( b ) The chromatin locus is visualized by Cherry-LacI staining. Cells were co-transfected with YFP-LacI and CFP-NDR-FL or with YFP-LacI-HP1α and CFP-NDR1 or its truncation mutants. YFP-LacI does not recruit CFP-NDR1 to the locus, whereas YFP-LacI-HP1α can efficiently recruit CFP-NDR1 to the chromatin locus. Cells co-transfected with YFP-LacI-HP1α and CFP-NDR1-ΔN or CFP-NDR1-ΔC shows accumulation at the HP1α containing locus. Scale bar, 10 μm. Full size image NDR1 kinase phosphorylates HP1α in vitro We next addressed the role of NDR kinase in HP1α phosphorylation employing in vitro kinase assays. Recombinant NDR1 kinase was used in the kinase assay with glutathione S -transferase (GST), GST-HP1α-wild type (WT), GST-HP1α-1-66aa, GST-HP1α-67-119aa, GST-HP1α-1-119aa and GST-HP1α-120-191aa as substrates ( Fig. 3a ). HP1α constructs with the CD and/or the hinge domain (region spanning 1–119 amino acids), but not the CSD (120–191 amino acids), could be efficiently phosphorylated by NDR1 kinase ( Fig. 3a ). Autophosphorylation of recombinant NDR1 was also observed; this was especially prominent in the absence of relevant substrates (120–191 amino acids). Similarly, NDR kinase purified from HEK 293 cells exhibited similar ability to modify HP1α ( Supplementary Fig. 2a ). 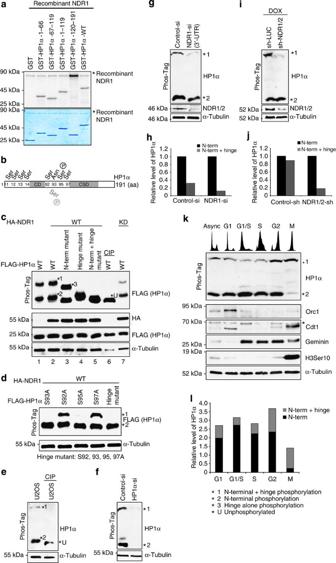Figure 3: NDR kinase phosphorylates HP1α. (a)In vitrokinase assay using recombinant NDR1 kinase and GST or GST-HP1α-WT or truncation mutants 1–66, 67–119, 1–119 and 120–191 as substrates. Coomassie-stained gel is shown below for the substrates. (b) Schematic representation of the various phosphorylation sites on human HP1α. Note that the serine 93 of mouse HP1α is substituted with asparagine in human. (c) Phos-tag PAGE analysis of lysates from cells transfected with FLAG-mHP1α with HA-NDR1 kinase or HA-NDR1-K118A or without either kinase. Two forms of HP1α, faster migrating form (*2) and slower migrating form (*1) are discernible in WT-HP1α. CIP treatment shows the mobility of dephosphorylated form. Phos-tag PAGE analysis of lysates expressing HA-NDR1 with FLAG-mHP1α-N-terminal mutant (S11–14A) represents a slower migrating hinge-alone phosphorylated form (*3) and a faster migrating unphosphorylated form (*U). The hinge mutant only shows faster migrating form (*2). α-Tubulin is shown as a loading control in regular SDS–PAGE. (d) Phos-tag PAGE analysis of lysates expressing HA-NDR1 along with single point mutants in the hinge region (S92A, S93A, S95A and S97A) of mouse HP1α and the combination of all (hinge mutant). (e) Phos-tag PAGE analysis of U2OS lysates treated with phosphatase followed by immunoblot analysis using HP1α antibody. (f) Phos-tag PAGE analysis of lysates from HP1α siRNA-treated cells followed by immunoblot analysis using HP1α antibody. (g,h) Phos-tag PAGE analysis of lysates from NDR-depleted cells using siRNA or shRNA (i,j) approach. Note the slower migrating mitotic-specific phosphorylated form of HP1α is reduced on NDR1/2 depletion. (k) Phos-tag PAGE analysis of lysates from U2OS cells synchronized at different stages of the cell cycle and immunoblot analysis with HP1α antibodies to detect endogenous HP1α. Note the slower migrating form is predominantly present during G2 and mitosis. Flow cytometry profile is provided at the top of the panel. Orc1 (present predominantly during G1); Cdt1 (present during G1, phosphorylated during M); geminin (present in post-G1 cells) and histone 3 phosphorylated at serine 10 (mitosis specific) are shown in regular SDS–PAGE. (l) Quantification of the relative levels of N-terminal and N-terminal+hinge phosphorylation of HP1α during different stages of the cell cycle based on the immunoblot ink. Figure 3: NDR kinase phosphorylates HP1α. ( a ) In vitro kinase assay using recombinant NDR1 kinase and GST or GST-HP1α-WT or truncation mutants 1–66, 67–119, 1–119 and 120–191 as substrates. Coomassie-stained gel is shown below for the substrates. ( b ) Schematic representation of the various phosphorylation sites on human HP1α. Note that the serine 93 of mouse HP1α is substituted with asparagine in human. ( c ) Phos-tag PAGE analysis of lysates from cells transfected with FLAG-mHP1α with HA-NDR1 kinase or HA-NDR1-K118A or without either kinase. Two forms of HP1α, faster migrating form (*2) and slower migrating form (*1) are discernible in WT-HP1α. CIP treatment shows the mobility of dephosphorylated form. Phos-tag PAGE analysis of lysates expressing HA-NDR1 with FLAG-mHP1α-N-terminal mutant (S11–14A) represents a slower migrating hinge-alone phosphorylated form (*3) and a faster migrating unphosphorylated form (*U). The hinge mutant only shows faster migrating form (*2). α-Tubulin is shown as a loading control in regular SDS–PAGE. ( d ) Phos-tag PAGE analysis of lysates expressing HA-NDR1 along with single point mutants in the hinge region (S92A, S93A, S95A and S97A) of mouse HP1α and the combination of all (hinge mutant). ( e ) Phos-tag PAGE analysis of U2OS lysates treated with phosphatase followed by immunoblot analysis using HP1α antibody. ( f ) Phos-tag PAGE analysis of lysates from HP1α siRNA-treated cells followed by immunoblot analysis using HP1α antibody. ( g , h ) Phos-tag PAGE analysis of lysates from NDR-depleted cells using siRNA or shRNA ( i , j ) approach. Note the slower migrating mitotic-specific phosphorylated form of HP1α is reduced on NDR1/2 depletion. ( k ) Phos-tag PAGE analysis of lysates from U2OS cells synchronized at different stages of the cell cycle and immunoblot analysis with HP1α antibodies to detect endogenous HP1α. Note the slower migrating form is predominantly present during G2 and mitosis. Flow cytometry profile is provided at the top of the panel. Orc1 (present predominantly during G1); Cdt1 (present during G1, phosphorylated during M); geminin (present in post-G1 cells) and histone 3 phosphorylated at serine 10 (mitosis specific) are shown in regular SDS–PAGE. ( l ) Quantification of the relative levels of N-terminal and N-terminal+hinge phosphorylation of HP1α during different stages of the cell cycle based on the immunoblot in k . Full size image NDR kinase phosphorylates HP1α in vivo HP1α has several predicted phosphorylation sites in the N terminus and within the hinge region. Recent studies have demonstrated that mammalian HP1α is phosphorylated at the N-terminal and hinge region [14] , [30] , [45] . Here we selected several putative serine residues of mammalian HP1α based on the phosphosite predictions and evaluated the in vivo phosphorylation status of these residues [46] ( Fig. 3b ). To demonstrate in vivo phosphorylation as well as to map the sites of phosphorylation within HP1α by NDR1 kinase, we co-transfected FLAG-tagged WT or several different point mutants (substitutions of serine to alanine of predicted phosphorylation site at the N-terminal and hinge region) of mouse HP1α and human HA-NDR1 in U2OS cells. The lysates were analysed by phos-tag polyacrylamide gel electrophoresis (PAGE). Phos-tag forms a complex with Mn +2 and traps R-OPO 3 −2 ; this enhances the mobility shifts of phosphorylated proteins [47] . WT-HP1α was highly phosphorylated in cells co-transfected with NDR kinase in vivo with two distinct phosphorylation patterns ( Fig. 3c , lane 2, see *1 and *2). Both the forms were sensitive to calf intestinal phosphatase (CIP) treatment and produce a faster migrating non-phosphorylated form of HP1α ( Fig. 3c , lane 6, *U). In the absence of NDR1 kinase, the slower migrating phosphorylated band (*1) of HP1α was somewhat reduced ( Fig. 3c , lane 1). The co-transfection with a kinase-deficient mutant form of NDR1 (K118A) also showed reduced phosphorylation of HP1α ( Fig. 3c , lane 7). To further map the residues on HP1α that are phosphorylated by NDR kinases, we used full-length HP1α mutants containing amino-acid substitutions that should result in a non-phosphorylatable N terminus (N-terminal mutant, serine at positions 11, 12, 13 and 14 were substituted with alanine) or non-phosphorylatable hinge region (hinge mutant, serine at positions 92, 93, 95 and 97 were substituted with alanine) or a combination of both as well as the single point mutants of N-terminal (S11A, S12A, S13A and S14A) and hinge region (S92A, S93A, S95A and S97A). An HP1α mutant where all the serines at the N-terminal (S11, 12, 13 and 14A) and at the hinge (S92, 93, 95 and 97A) were substituted with alanines, a complete loss of phosphorylation was observed ( Fig. 3c , lane 5). Further, mobility of this mutant HP1α was equivalent to that of the WT-HP1α treated with CIP ( Fig. 3c , compare lane 5 with 6). The faster migrating band of N-terminal mutant ( Fig. 3c , lane 3) showed mobility similar to the unphosphorylated form (*U, Fig. 3c , lane 6). Also, the slower migrating form in the N-terminal mutant-transfected cells (*3) migrated faster compared with the slower migrating form in WT-transfected cells (*1), ( Fig. 3c , compare lane 2 with 3). Further, dissection of the N-terminal end revealed that the point mutant, S14A the predominant phosphorylation site ( Supplementary Fig. 2b , lane 4) showed similar profile to that of the N-terminal mutant ( Supplementary Fig. 2b , lane 5). Further analysis using the hinge region mutant (S92A, S93A, S95A and S97A) co-transfected with NDR kinase revealed a loss of the slower migrating form altogether ( Fig. 3c , lane 4). However, these mutants showed no change in the mobility of the faster migrating form, suggesting that changes in the phosphorylation within the hinge region do not affect the N-terminal phosphorylation (Fig. 3d ). Both S93A and S95A mutations of the hinge region resulted in disappearance of slower migrating form, suggesting that these two sites represent the primary phosphorylation sites of NDR1 in the hinge region ( Fig. 3d and Supplementary Fig. 2c ). Interestingly, although human and mouse HP1α are highly conserved (~99%), serine 93 of mouse HP1α is substituted with asparagine in human ( Fig. 3b ). We therefore suggest that the predominant site of phosphorylation within the hinge region of human HP1α is serine 95 ( Fig. 3d ). A fainter slower migrating form can also be observed on overexposure in S95A mutant perhaps owing to the presence of intact serine 93 in this mutant ( Supplementary Fig. 2c ). These above results revealed that the fast migrating form (*2 in Fig. 3c,d ) represented HP1α phosphorylated at the N-terminal region alone, whereas the slower migrating form (*1) denoted HP1α phosphorylated in the hinge region in addition to the N terminus. Immunoblots using HP1α antibody to detect endogenous HP1α on Phos-tag gels revealed two forms of HP1α in human cells similar to our observations when mouse HP1α was transiently expressed ( Fig. 3e , U2OS, asynchronous). Furthermore, phosphatase treatment showed that both the forms collapsed to an unphosphorylated form ( Fig. 3e ). Further, it was evident that the N-terminal domain was constitutively phosphorylated, since unphosphorylated form of HP1α was never detectable. Analysis of HP1α small interfering RNA (siRNA)-treated extracts further confirmed the specificity of both the phosphorylated forms ( Fig. 3f ). To address whether NDR1 kinase phosphorylates HP1α in vivo , we next examined the status of phosphorylation of HP1α in cells lacking NDR kinase. Phos-tag electrophoresis analysis revealed that in NDR kinase-depleted cells (using both siRNA and short hairpin RNA (shRNA)), there was a significant reduction in the slower migrating band of HP1α (*1) without any significant alteration in the faster migrating band (*2; Fig. 3g–j ). The decrease in the phosphorylation at the hinge region (slower migrating band) of HP1α on NDR depletion further confirmed that NDR kinase is responsible for phosphorylating HP1α within the hinge region in vivo ( Fig. 3g–j ). While the in vitro data demonstrated that NDR kinase could also phosphorylate HP1α at the N-terminal domain, no significant and consistent changes in the N-terminal phosphorylation of HP1α were observed in NDR1/2-depleted cells. These results suggest that other kinases (in addition to NDR kinase) may phosphorylate HP1α at its N-terminus domain in vivo . We next examined whether phosphorylation of HP1α at specific serine residues at the N terminus and the hinge region are cell cycle regulated. During G1, G1/S, S and G2 phase, the faster migrating form representing the N-terminal phosphorylation of endogenous HP1α was predominant, whereas cells at G2 also showed increased levels of the slower migrating form of HP1α representing phosphorylation at the N terminus+hinge regions ( Fig. 3k,l ). By mitosis, the slower migrating form represented the prominent form of HP1α in the cells ( Fig. 3k,l ). Interestingly, there was an increase in the levels of slower migrating form (N terminal+hinge) of HP1α in G2 and M phase with a concomitant decrease in the faster migrating form specifically during mitosis ( Fig. 3k,l ). In addition, we have also observed other migrating forms of HP1α in between form *1 and *2, especially in mitotic extracts ( Fig. 3k ). We believe that these represent other phosphorylated forms of HP1α that are present at lower levels. Similar observations, where we detect slower migrating forms during mitosis, were made in cells co-transfected with FLAG-HP1α and HA-NDR1 and synchronized at mitosis. In nocodazole-arrested cells expressing only the FLAG-HP1a, the slower migrating form was apparent in addition to the faster migrating one ( Supplementary Fig. 2d ). Contrary to the data obtained with endogenous HP1α (see Fig. 3k,l ), FLAG-HP1α-expressing prometaphase-arrested cells continued to show higher levels of N-terminal-alone phosphorylated faster migrating form of HP1α (the ratio of faster migrating (lower) versus slower migrating (upper) band in the absence of NDR1 is 1.85/1; Supplementary Fig. 2d ). We speculated that the cellular pool of NDR1 might be limiting for the cells to phosphorylate the hinge domain of most of the exogenously expressed HP1α. To test this, we co-expressed both HP1α and NDR1, and in prometaphase cells the ratio of the slower migrating form to the faster migrating form was found altered with increased levels of the slower migrating form being apparent (the ratio changed to 1/1.29; Supplementary Fig. 2d ). On the basis of all the data, we conclude that during mitosis most of the cellular HP1α undergoes hinge-specific phosphorylation by NDR kinase. S95 phospho-HP1α localizes to centromeres during mitosis To address the functional relevance of the cell cycle-regulated hinge-specific phosphorylation of HP1α in human cells, we have generated HP1α-S95-specific phospho-antibody. Depletion of HP1α using HP1α-specific siRNA oligonucleotides followed by immunoblot analysis in HeLa whole-cell extracts using HP1α antibody as well as S95-specific phospho-antibody revealed that the S95 antibody detected HP1α only in control cells but not in HP1α-depleted cells ( Fig. 4a ). Further, immunoblot analysis in cell lysates treated with CIP using the S95 antibody showed significantly reduced signal further confirming the specificity of this antibody ( Fig. 4a ). We have shown that HP1α is constitutively phosphorylated in vivo . The HP1α antibody that can recognize both phosphorylated and unphosphorylated forms recognizes the phosphorylated HP1α more prominently than the unphosphorylated form ( Fig. 4a ). We next examined the cellular abundance of hinge-phosphorylated form of HP1α during different stages of the cell cycle using S95 specific-antibody. Hinge-phosphorylated form of HP1α was most prominent during G2 and mitosis ( Fig. 4b ) with reduced levels during G1 phase, corroborating our previous results ( Fig. 3k ). In contrast, the HP1α antibody showed reduced signals during mitosis, because the overall levels of HP1α during G1/S seem to be much higher than during mitosis. Furthermore, phos-tag immunoblot analysis in M phase and G1-synchronized cell extracts revealed that S95 antibody detected the N-terminal+hinge phosphorylated form of HP1α (slower migrating form *1; Fig. 4c ). S95 antibody occasionally detected a band that has the mobility in between the two phosphorylated forms. This may represent the hinge-only phosphorylated form. These results further confirm that the slower migrating form of HP1α present during G2 and mitosis is phosphorylated predominantly at serine 95. 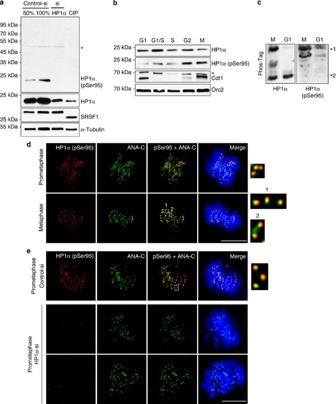Figure 4: Hinge-specific phosphorylated form of HP1α localizes at kinetochores during early mitosis. (a) Immunoblot analysis of lysates using HP1α-S95 phospho-antibody (Ab) from HeLa cells that are depleted of HP1α using siRNA and treated with CIP on regular SDS–PAGE. SRSF1 is shown as a control. (b) Immunoblot analysis of lysates from different stages of the cell cycle using HP1α-S95 phospho-Ab on regular SDS–PAGE. Note the increased signal with S95 antibody during G2 and mitosis. (c) Phos-tag PAGE analysis of lysates from cells synchronized at mitosis (M) or G1 phase and immunoblot analysis with HP1α and HP1α-S95 phospho-Abs. Note that S95 phospho-Ab does not detect the faster form of HP1α. (d) Immunofluorescence localization of hinge-specific phosphorylation of HP1α using S95 phospho-Ab (red) along with centromere marker ANA-C (green) in human HeLa cells. Note the association of phosphorylated form of HP1α in the vicinity of centromeres in prophase and metaphase. Inset (5 × ) shows that the red signals are exterior to green, suggesting the presence of this modified form of HP1α at outer kinetochores. Scale bar, 10 μm. (e) Immunofluorescence using S95 and ANA-C antibodies in U2OS cells treated with control or HP1α siRNA. Note the loss of centromeric signal of S95 in HP1α siRNA-treated cells. Inset (5 × ) shows that the red signals are exterior to green. Scale bar, 10 μm. Figure 4: Hinge-specific phosphorylated form of HP1α localizes at kinetochores during early mitosis. ( a ) Immunoblot analysis of lysates using HP1α-S95 phospho-antibody (Ab) from HeLa cells that are depleted of HP1α using siRNA and treated with CIP on regular SDS–PAGE. SRSF1 is shown as a control. ( b ) Immunoblot analysis of lysates from different stages of the cell cycle using HP1α-S95 phospho-Ab on regular SDS–PAGE. Note the increased signal with S95 antibody during G2 and mitosis. ( c ) Phos-tag PAGE analysis of lysates from cells synchronized at mitosis (M) or G1 phase and immunoblot analysis with HP1α and HP1α-S95 phospho-Abs. Note that S95 phospho-Ab does not detect the faster form of HP1α. ( d ) Immunofluorescence localization of hinge-specific phosphorylation of HP1α using S95 phospho-Ab (red) along with centromere marker ANA-C (green) in human HeLa cells. Note the association of phosphorylated form of HP1α in the vicinity of centromeres in prophase and metaphase. Inset (5 × ) shows that the red signals are exterior to green, suggesting the presence of this modified form of HP1α at outer kinetochores. Scale bar, 10 μm. ( e ) Immunofluorescence using S95 and ANA-C antibodies in U2OS cells treated with control or HP1α siRNA. Note the loss of centromeric signal of S95 in HP1α siRNA-treated cells. Inset (5 × ) shows that the red signals are exterior to green. Scale bar, 10 μm. Full size image We next examined the localization of the hinge-specific phosphorylation of HP1α using affinity-purified S95 phospho-antibody. Co-immunolocalization using S95 antibody and centromere-specific antibody (ANA-C) in human cell lines, including HeLa cells ( Fig. 4d ) and U2OS cells ( Supplementary Fig. 3a ) demonstrated that the hinge-specific form of HP1α was present in the vicinity of the centromeres prominently during prometaphase. In most of the occasions, the S95 signal was located on the outer edge of the ANA-C (recognizing CENP-A) antibody-stained centromeres, reminiscent of kinetochore distribution (please see the insets in Fig. 4d,e ). Co-immunolocalization using S95 antibody and outer kinetochore-specific Mad1 in human HeLa cells further confirmed the kinetochore association of phosphorylated HP1α ( Supplementary Fig. 3e,f ). The kinetochore association of hinge-specific phosphorylated form of HP1α reduced further as the cells progressed through mitosis and was no longer evident during anaphase and telophase ( Supplementary Fig. 3a ). However, an antibody against HP1α that recognizes all the forms of HP1α detected HP1α at centric and pericentromeric heterochromatin throughout mitosis ( Supplementary Fig. 3d ). These results demonstrate that the S95-specific phosphorylated form of HP1α preferentially localizes at kinetochores during early mitosis and is lost from these sites as the cells progress through mitosis. Use of pre-immune serum as well as peptide block experiments confirmed the specificity of the antibody ( Supplementary Fig. 3b,c ). To further confirm the specificity of the S95 antibody, we carried out immunostaining using this antibody in U2OS cells treated with HP1α siRNA. Specific signals at the centromeres using S95 antibody were almost completely diminished in HP1α siRNA-treated cells but not in the control cells ( Fig. 4e ). Depletion of NDR kinase results in mitotic abnormalities To address the physiological relevance of NDR kinase-mediated phosphorylation of HP1α, we examined how NDR1 influences HP1α function in vivo . We conducted RNA interference-mediated knockdown of NDR using two siRNAs (siRNA against 3′-untranslated region (UTR) and coding region of NDR1) oligonucleotides as well as shRNA in human U2OS cell lines [48] . We achieved >70% knockdown of NDR (both by siRNA and shRNA treatment) and found that the cells lacking these kinases did not show significant alteration in the total cellular levels of HP1α and other HP1 isoforms ( Fig. 5a and Supplementary Fig. 4a ). Immunoblot with an antibody that detected both NDR1 and NDR2 in control and NDR1 si-treated cells indicated that depletion of NDR1 also reduces the levels of NDR2. Human genome contains two NDR genes, NDR1 and NDR2 . We have observed that both NDR1 and NDR2 kinases interact with one another ( Supplementary Fig. 4b ) and therefore there seems to be co-operativity between these two kinases. We have also observed that NDR1 homodimerizes/homomultimerizes ( Supplementary Fig. 4c ). We are currently investigating the homo-di/multimerization of NDR1 and its heteromerization with NDR2 and its impact on the functionality of these kinases. 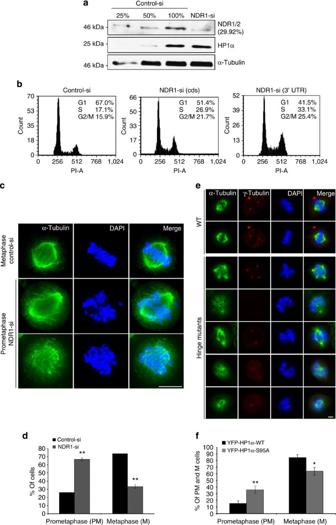Figure 5: Hinge-specific phosphorylation of HP1α is required for accurate chromosome alignment and mitotic progression. (a) Immunoblot analysis of lysates from cells that are depleted of NDR kinase using siRNA. The upper panel denotes the percentage of whole-cell extracts (WCE) loaded in control; the knockdown represents 100% WCE. Note that >70% knockdown of NDR1 was achieved. (b) Flow cytometry in control and NDR-depleted cells using two different siRNA targeting the coding region (cds) and 3′-UTR of NDR1. (c) Immunofluorescence analysis using α-tubulin antibodies to study mitotic phenotype. (d) Note an increase in prometaphase population on NDR depletion. Error bars represent s.d. of three independent experiments. Statistical significance was determined by Student’st-test. Mean±s.d., *P<0.05, **P<0.01 and ***P<0.001. Scale bar, 10 μm. (e) Overexpression of FLAG-S95A and hinge mutant (S92, S93, 95, 97A) of mouse HP1α in human U2OS cells and immunofluorescence analysis using α- and γ-tubulin. Note mitotic abnormalities in cells expressing mutants. Scale bar, 10 μm. (f) Transient transfection of YFP-HP1α-WT and YFP-HP1α-S95A mutant, followed by statistical analysis of mitotic population. Note the accumulation of prometaphase stage in cells expressing YFP-HP1α-S95A mutants. Error bars represent s.d. of three independent experiments. Statistical significance was determined by Student’st-test. Mean±s.d., *P<0.05 and **P<0.01. Scale bar, 10 μm. Figure 5: Hinge-specific phosphorylation of HP1α is required for accurate chromosome alignment and mitotic progression. ( a ) Immunoblot analysis of lysates from cells that are depleted of NDR kinase using siRNA. The upper panel denotes the percentage of whole-cell extracts (WCE) loaded in control; the knockdown represents 100% WCE. Note that >70% knockdown of NDR1 was achieved. ( b ) Flow cytometry in control and NDR-depleted cells using two different siRNA targeting the coding region (cds) and 3′-UTR of NDR1. ( c ) Immunofluorescence analysis using α-tubulin antibodies to study mitotic phenotype. ( d ) Note an increase in prometaphase population on NDR depletion. Error bars represent s.d. of three independent experiments. Statistical significance was determined by Student’s t -test. Mean±s.d., * P <0.05, ** P <0.01 and *** P <0.001. Scale bar, 10 μm. ( e ) Overexpression of FLAG-S95A and hinge mutant (S92, S93, 95, 97A) of mouse HP1α in human U2OS cells and immunofluorescence analysis using α- and γ-tubulin. Note mitotic abnormalities in cells expressing mutants. Scale bar, 10 μm. ( f ) Transient transfection of YFP-HP1α-WT and YFP-HP1α-S95A mutant, followed by statistical analysis of mitotic population. Note the accumulation of prometaphase stage in cells expressing YFP-HP1α-S95A mutants. Error bars represent s.d. of three independent experiments. Statistical significance was determined by Student’s t -test. Mean±s.d., * P <0.05 and ** P <0.01. Scale bar, 10 μm. Full size image Flow cytometry analysis of NDR1-depleted cells demonstrated a decrease in G1 phase with a concomitant increase in G2/M population ( Fig. 5b and Supplementary Fig. 4d ), suggesting that NDR kinase is required for cell cycle progression. We have observed significant loss of hinge-specific mitotic phosphorylation of HP1α in NDR1-depleted cells ( Fig. 3g–j ), suggesting that this post-translational modification may have a crucial function in mitotic progression. Phenotypic analysis of mitotic cells demonstrated that in control cells, a total of 26±0.02% (for control siRNA-treated cells) and 25±11.6% (shLUC control cells) of mitotic cells were present in prometaphase stage (± denotes s.d. of the mean from three independent experiments). We observed an increase in prometaphase population (67±2% for NDR1 siRNA- and 60±15.7% for NDR shRNA-treated cells; ± denotes s.d. of the mean from three independent experiments) with a concomitant decrease in metaphase populations in the NDR kinase-depleted cells ( Fig. 5c,d and Supplementary Fig. 4e,f ). These results indicate that NDR1-depleted cells show defects in chromosome alignment and therefore display defects in mitotic progression. Since we observed mitotic defects with cells arrested during prometaphase and loss of hinge-specific phosphorylation of HP1α on NDR-depletion, we examined whether phosphorylation of HP1α is required for mitotic progression. To address the role of phosphorylation within the hinge region of HP1α, we conducted overexpression of the non-phosphorylatable mutants (FLAG-tagged mouse HP1α mutated at S95A or S92, 93, 95, 97A) and examined its effect on mitosis. We observed variable chromosome alignment defects in cells expressing hinge mutants in comparison with controls ( Fig. 5e ). Further, we have also observed aberrant spindle morphology. Defective spindles could also cause delay in the alignment of chromosomes and the extent of these defects could be attributed to the penetrance of the phenotype. Moreover, transient overexpression of YFP-HP1α-S95A mutant significantly increased the prometaphase population over cells expressing WT-HP1α ( Fig. 5f ). In control cells we observed 16±4% of prometaphase, 84±4% of metaphase, in contrast, S95A expressing cells showed 36±5% of cells in prometaphase and 64±5% in metaphase (± denotes s.d. of the mean from three independent experiments). Therefore, the HP1α-S95A hinge mutants of HP1α phenocopy NDR depletion, further supporting the role of NDR1-mediated phosphorylation of HP1α in proper chromosome alignment and hence mitotic progression perhaps mediating the prometaphase to metaphase transition. We also depleted endogenous NDR1 from HeLa cells followed by the immunolocalization of hinge phosphorylated HP1α at the mitotic centromere using S95-specific phospho-antibody. We observed a reduction of phospho-HP1α at mitotic centromeres on NDR1 depletion ( Supplementary Fig. 4g ), indicating the NDR1-mediated phosphorylation of HP1α is required for the localization of HP1α to centromeres. We next evaluated the localization of YFP-HP1α-S95A mutant as well as YFP-HP1α-S95E mutant in cells where the endogenous HP1α (using 3′-UTR-specific siRNAs) was depleted. Immunoblots demonstrated that 3′-UTR-specific siRNA treatment resulted in the reduction of endogenous HP1α but did not alter the overall levels of YFP-tagged HP1α mutants ( Supplementary Fig. 5a ). YFP-HP1α-S95A localization to the mitotic centromeres was reduced in the absence of endogenous HP1α ( Supplementary Fig. 5b ). YFP-HP1α-S95A associated with centromeres only in cells that contained intact endogenous HP1α. This is explained by our observation that the mutants can efficiently interact with the WT-HP1α and therefore can be recruited to the centromeres by virtue of their association with the WT-HP1α ( Supplementary Fig. 5c ). On the other hand, the phospho-mimetic mutant of HP1α (YFP-HP1α-S95E) bound to mitotic centromeres in the presence or absence of endogenous HP1α ( Supplementary Fig. 5b ). These results suggest that the mitotic defects in NDR-depleted cells may be due to changes in the phosphorylation status of HP1α, since reduced phosphorylation in the hinge domain of HP1α reduced its ability to localize to centromeric region. Phospho S95 facilitates Sgo1 binding to mitotic centromeres Next we were interested to understand the role of hinge phosphorylation of HP1α in mitotic progression. HP1-mediated targeting of the Sgo1 to mitotic centromeres is required for centromeric sister chromatid cohesion [28] . We examined the localization of Sgo1 to centromeres during mitosis in NDR1-siRNA- and HP1α-siRNA-treated cells. We have systematically counted (>150 cells) and looked for centromeric staining of Sgo1 in prometaphase cells. Presence of clear puncta was categorized as positive, whereas diffuse signal with no enrichment at the centromeres were categorized as negative. We observed a significant decrease in the localization of Sgo1 to mitotic centromeres in cells lacking NDR1 as well as HP1α (around 91±5% cells showed Sgo1 staining on mitotic centromere in control siRNA-treated cells, whereas 44±5.6% for NDR1 siRNA- and 16±1.1% for HP1α siRNA-treated cells. (± denotes s.d. of the mean from three independent experiments; Fig. 6a,e ; Supplementary Fig. 5d ). To address whether the hinge-specific phosphorylation of HP1α facilitates the Sgo1 localization to mitotic centromeres, we individually depleted either NDR1 kinase or HP1α (utilizing siRNA oligonucleotides targeting the 3′-UTR of NDR1 and HP1α, respectively) in cells stably expressing YFP-HP1α-WT, YFP-HP1α-S95A or YFP-HP1α-S95E. Depletion of NDR1 or HP1α in YFP-HP1α-S95A background continued to show lack of Sgo1 association to mitotic centromeres (91±5% in controls, 41±12.3% for NDR1 siRNA- and 21±4.7% for HP1α siRNA-treated cells; ± denotes s.d. of the mean. Data were calculated from triplicates; Fig. 6c,e ; Supplementary Fig. 5d ). We have observed similar loss of Sgo1 staining from centromeres in YFP-HP1α-WT cells on NDR1 depletion (96±1.5% in controls, 51±6.5% for NDR1 siRNA-treated cells; ± denotes s.d. of the mean. Data were calculated from triplicates; Fig. 6b,e ) Interestingly, in NDR1 or HP1α-depleted cells expressing YFP-HP1α-S95E, the number of mitotic cells that decorated Sgo1 at centromeres increased significantly (75±5.8% for NDR1 siRNA- and 69±8% for HP1α siRNA-treated cells; ± denotes s.d. of the mean. Data were calculated from triplicates; Fig. 6d,e ; Supplementary Fig. 5d ). Similarly, localization of Sgo1 at mitotic centromeres was partially rescued in endogenous NDR1-depleted cells (using 3′-UTR-specific siRNA) that were stably expressing HA-NDR1, but not in cells expressing vector alone or the kinase-deficient NDR1 ( Fig. 6f ). These results demonstrate that NDR1 kinase (and perhaps NDR1 kinase-mediated phosphorylation of HP1α at the hinge region) directly/indirectly facilitates the localization of Sgo1 to mitotic centromeres. It is well established that the recruitment of Sgo1 to mitotic centromeres is crucial for chromosome segregation [28] . We demonstrate that NDR depletion causes significant reduction in HP1α phosphorylation, defects in Sgo1 localization to centromeres and mitotic abnormalities. On the basis of these results, we propose that the hinge phosphorylation of HP1α during mitosis by NDR1 facilitates the proper loading of Sgo1 to centromeres ( Fig. 7 ). 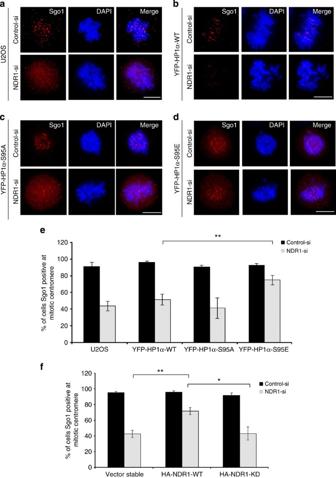Figure 6: Hinge-specific phosphorylation of HP1α facilitates Sgo1 binding to mitotic centromeres. (a) Immunofluorescence using Sgo1 antibody in NDR1-depleted cells in U2OS cells; (b) YFP-HP1α-WT-; (c) YFP-HP1α-S95A- and (d) YFP-HP1α-S95E-expressing cells. DNA is counterstained with 4',6-diamidino-2-phenylindole (DAPI). Scale bar, 10 μm. (e) Quantification of the presence of Sgo1 at mitotic centromeres (prometaphase stage). Note the increased binding of Sgo1 to centromeres in NDR1-depleted YFP-HP1α-S95E-expressing cells. Error bars represent s.d. of three independent experiments. Statistical significance was determined by Student’st-test. Mean±s.d., *P<0.05 and **P<0.01. (f) Quantification of Sgo1 presence (Sgo1+) at mitotic centromeres in cells expressing empty vector, HA-NDR1-WT or HA-NDR1-KD (K118A) and lacking NDR1 kinase. Error bars represent s.d. of three independent experiments. Statistical significance was determined by Student’st-test. Mean±s.d., *P<0.05 and **P<0.01. Note the rescue of Sgo1 signal at centromeres in HA-NDR1-expressing cells. Figure 6: Hinge-specific phosphorylation of HP1α facilitates Sgo1 binding to mitotic centromeres. ( a ) Immunofluorescence using Sgo1 antibody in NDR1-depleted cells in U2OS cells; ( b ) YFP-HP1α-WT-; ( c ) YFP-HP1α-S95A- and ( d ) YFP-HP1α-S95E-expressing cells. DNA is counterstained with 4',6-diamidino-2-phenylindole (DAPI). Scale bar, 10 μm. ( e ) Quantification of the presence of Sgo1 at mitotic centromeres (prometaphase stage). Note the increased binding of Sgo1 to centromeres in NDR1-depleted YFP-HP1α-S95E-expressing cells. Error bars represent s.d. of three independent experiments. Statistical significance was determined by Student’s t -test. Mean±s.d., * P <0.05 and ** P <0.01. ( f ) Quantification of Sgo1 presence (Sgo1+) at mitotic centromeres in cells expressing empty vector, HA-NDR1-WT or HA-NDR1-KD (K118A) and lacking NDR1 kinase. Error bars represent s.d. of three independent experiments. Statistical significance was determined by Student’s t -test. Mean±s.d., * P <0.05 and ** P <0.01. Note the rescue of Sgo1 signal at centromeres in HA-NDR1-expressing cells. 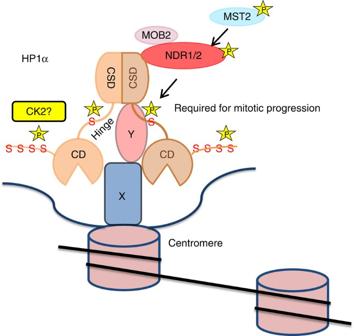Figure 7: Phosphorylation of HP1α is required for accurate mitotic progression. Model depicting the association of phosphorylated HP1α within the N terminus associating with the chromatin mark H3trimethyl-K9. NDR kinase binds to the CSD of HP1α and phosphorylates the hinge domain during G2/M stages of cell cycle that in turn may facilitate its association with centromeric proteins (X and Y represent unknown proteins at centromere; Sgo1 is a good candidate for Y) and accurate chromosome alignment and mitotic progression. Stars represent phosphorylation sites. Full size image Figure 7: Phosphorylation of HP1α is required for accurate mitotic progression. Model depicting the association of phosphorylated HP1α within the N terminus associating with the chromatin mark H3trimethyl-K9. NDR kinase binds to the CSD of HP1α and phosphorylates the hinge domain during G2/M stages of cell cycle that in turn may facilitate its association with centromeric proteins (X and Y represent unknown proteins at centromere; Sgo1 is a good candidate for Y) and accurate chromosome alignment and mitotic progression. Stars represent phosphorylation sites. Full size image HP1α, a heterochromatin-associated protein, facilitates the assembly of higher-order chromatin structure and plays key roles in various chromosome functions including sister chromatid cohesion and transcriptional gene silencing [27] . Similar to histones, HP1 isoforms are decorated with extensive post-translational modifications that are often linked with their biological functions [14] . In this study, we demonstrate that mammalian HP1α is constitutively phosphorylated within its N terminus and additional phosphorylation within the hinge domain becomes apparent as the cells progress from G2 to mitosis, and this modification is required for mitotic progression. HP1 has been shown to be required for accurate chromosome segregation in Drosophila embryos [49] , in fission yeast [24] , [50] as well as in mammalian cells [51] , [52] . HP1/Swi6 in fission yeast is required for the recruitment of cohesins to centromeres and the establishment of the centromeric histone H3 variant CENP-A Cnp1 , which is crucial to regulate chromosome alignment and segregation [1] , [24] , [53] , [54] , [55] . The targeting of HP1α to centromeric heterochromatin occurs through two independent mechanisms. In interphase nuclei, the trimethylated lysine 9 of histone H3 is important for targeting HP1α to centromeric heterochromatin [3] , [4] and the phosphorylation at N-terminal serine residues of HP1α enhances the interaction of HP1α with trimethylated H3K9 (ref. 30 ). However, during mitosis phosphorylation by Aurora B kinase at serine 10 of H3 (H3S10) disrupts this interaction and releases most of the HP1α from chromatin except at centromeres [56] . Therefore, a CD-independent event operates to recruit HP1α to mitotic centromeres, involving an interaction between chromosomal passenger protein INCENP and HP1 CSD through the PXVXL/I motif [57] , [58] . Characterization of centromeric proteins that specifically associate with the hinge-phosphorylated HP1α at kinetochores will be a goal for future studies. A recent study by Hiragami-Hamada et al. [30] described a role for the N-terminal phosphorylation of HP1α in enhanced chromatin binding. Although it is largely believed that CKII is the kinase that phosphorylates HP1α, in vivo data obtained on CKII depletions show no effect on HP1α phosphorylation [30] . We demonstrate that mammalian HP1α is a mitotic substrate for NDR kinase. Using immunoprecipitation experiments we have demonstrated the interaction of NDR1 kinase and HP1α. We were, however, unable to detect a direct interaction between HP1α and NDR1. This is not surprising since the interaction between kinase and its substrates are known to be highly transient in nature and have strong dependency on the cellular context [59] , [60] . However, HP1α-W174A, a chromoshadow domain mutant that has lost its ability to bind PXVXL/I ligands showed almost complete loss of interaction with NDR1 kinase. The NDR family of serine threonine kinases, exist as four related kinases in human cells: NDR1, NDR2, LATS1 (large tumour suppressor-1) and LATS2, and all of them play key roles in many vital cellular processes, including cell growth, proliferation and differentiation, G1/S transition, centrosome duplication, mitotic chromosome alignment, mitotic exit and cytokinesis [33] . The cell cycle protein p21 is the only known in vivo substrate identified for NDR kinase in human cells [40] . Recent work demonstrated that NDR1 kinase is required for accurate chromosome alignment [41] . Further, it was demonstrated that the activation of NDR by the upstream pathway comprising MST2 kinase, Furry and Mps-one-binding, determine the accuracy of chromosome alignment on the metaphase plates [41] . We have observed that in the NDR1-depleted cells, chromosomes failed to align at the metaphase plate with cells accumulating in prometaphase. Furthermore, a small population of cells showed spindle abnormalities consistent with the previously described role of NDR1 in maintaining spindle integrity and centrosome structure [61] . Work by Mizuno and co-workers have demonstrated that the kinase activity of NDR1 is required for chromosome alignment [41] . However, the substrates that are phosphorylated by NDR1 kinase that may drive accurate chromosome alignment had yet to be identified. We have now demonstrated that HP1α is a mitotic substrate for NDR1 kinase and that the phosphorylation of HP1α is crucial for chromosome alignment and mitotic progression. Our present data indicate that NDR1 kinase is responsible for the G2/M phosphorylation within the hinge region of HP1α, as depletion of NDR1 results in significantly reduced phosphorylation of HP1α within the hinge region. This is consistent with the fact that the kinase activity of NDR1 was reported to be enhanced about 4.4-fold in mitotic cells as compared with S-phase cells [41] . We observe that the hinge-specific phosphorylated form of HP1α localizes at kinetochores predominantly during prophase and prometaphase and is subsequently released from these sites during later stages of mitosis. Further, we observed prometaphase arrest in cells that were either depleted of NDR1 or in which the HP1α-S95A hinge mutant of HP1α was overexpressed. These results suggest that the hinge-specific phosphorylation of HP1α is crucial for mitotic progression. Furthermore, NDR1 or HP1α depletion caused reduced association of Sgo1 to centromeres. Sgo1 has been shown to protect centromeric sister chromatid cohesion during prophase [62] . Our results demonstrate that the phosphorylated form of HP1α facilitates the localization of Sgo1 to the mitotic centromeres. We also observed that the HP1α-S95A mutant failed to localize to the centromeres suggesting that the phosphorylated form of HP1α may tether Sgo1 directly or indirectly to the mitotic centromeres. HP1α has previously been implicated in promoting Sgo1 centromeric localization [28] . However, a recent study has suggested that a Sgo1 mutant deficient in HP1 binding is functional in sister chromatid cohesion and localizes to centromeres [58] . Our data support a role for NDR1-mediated hinge-specific phosphorylation of HP1α in facilitating Sgo1 binding to centromeres directly or indirectly. In addition, several redundant mechanisms are known to enable the Sgo1 targeting to mitotic centromeres [58] . Earlier studies reported defects in mitotic chromosome alignment and in the activation of Aurora B on NDR1 depletion [41] , [63] . It is a possibility that the hinge-specific phosphorylation of HP1α protein, in addition to governing Sgo1 binding to centromeres, also modulates the Aurora B activity to promote accurate and faithful mitotic chromosome alignment and segregation. Activation of Aurora B, as well as its positioning at heterochromatin has been shown to require INCENP [64] , [65] . Furthermore, Aurora B associates with the C terminus of INCENP, while the hinge region of HP1α binds to the N terminus of INCENP [65] , [66] . Phosphorylation of HP1α at the hinge region might modulate the interaction of HP1α with Sgo1 and perhaps INCENP at centromeres ( Fig. 7 ). It is likely that the lack of NDR1 kinase might affect multiple pathways that prevent Sgo1 association to mitotic centromeres. Our data support a role for NDR-mediated hinge-specific phosphorylated HP1α in recruiting Sgo1 directly or indirectly to the mitotic centromeres. However, a possibility of HP1α-independent role of NDR1 in regulating Sgo1 can also be considered. The role of Sgo1 in cohesion protection has been shown to be antagonized by the mitotic kinase Plk1 and aurora B [67] . On the other hand, the kinase activity of Aurora B was increased in cells depleted of NDR1 or MST1, an upstream kinase of NDR1 (ref. 63 ). Moreover, similar to NDR1 depletion, depletion of MST1 also resulted in mitotic arrest with unaligned mitotic chromosomes and the activation of the Mad2- and BubR1-dependent spindle checkpoint response [63] . Therefore, it is possible that depletion of NDR1 hyperactivates Aurora B, which in turn destabilizes the Sgo1 on mitotic chromosome. Similarly, depletion of either Mad2 or Aurora B has been shown to abrogate the mitotic arrest phenotype induced by Bub1 and Sgo1 depletion [68] . Future studies will focus on the role of NDR1 kinase and phosphorylated HP1α in the loading of Sgo1 to the centromeres. Cell culture and generation of stable cell lines Cell lines used in this study were obtained from the American Type Culture Collection grown in DMEM containing high glucose, supplemented either with 10% fetal bovine serum (FBS; Hyclone for U2OS) or reduced tetracyclin FBS (Tet system approved FBS; Clontech for 2-6-3 CLTon). Cells were transfected with Lipofectamine 2000 (Invitrogen) as per the manufacturers’ protocol. For generation of stable tetracycline-inducible cell lines expressing tetracyclin-regulated shRNA against NDR1 and 2, U2OS cells-TetON were transfected with pTER-NDR1/2 and pTER-Luciferase (control shRNA; kind gift from Brian A Hemmings). Cell clones were selected and maintained by growing them in the presence of 200 μg ml −1 zeocin and 200 μg ml −1 hygromycin. YFP-HP1α-WT, mS95A and mS95E cell lines were generated by transfecting the corresponding constructs in U2OS cell lines followed by selecting and maintaining them in the media containing G418 (Invitrogen). Lentiviral expression system was used for stable integration of HA-NDR1-WT or HA-NDR1-KD or empty vector in U2OS cells. Cell clones were selected by growing them in the presence of puromycin (2 μg ml −1 ). Plasmids and antibodies For different experiments, WT human NDR1 complementary DNA was cloned in pCGN ( Xba I/ Bam HI) or pCGT ( Xba I/ Bam HI). The C-terminal (amino acids 1–84, 1–100, 1–175 and 1–225) and N-terminal (amino acids 85–435, 142–465 and 188–465) deletion mutants were cloned in pCGT or pECFP-C1 vectors. The coding region of human NDR1 was also cloned into pECFP-C1 vector. The coding region of human HP1α was cloned into pEYFP-LacI vector (modified from pEGFP-LacI; kindly provided by Miroslav Dundr) [69] . The YFP-tagged WT (1–191 amino acids) and truncated mutants (1–75, 81–191, 121–180 and 121–191 amino acids) of human HP1α were kindly provided by Yasushi Hiraoka [57] . GST-tagged WT and truncated mutants (1–66, 67–119, 1–119 and 120–191 amino acids) and FLAG-tagged WT mouse HP1α and its serine to alanine point mutants were the kind gifts from Pierre Chambon and Jun-ichi Nakayama, respectively. The antibodies used in this study were as follows: anti-T7 (Novagen 69522, 1:5,000), anti-HA (12CA5, 1:500) anti-HP1α (for western blot (WB), Chemicon MAB3446, 1:500 and for immunostaining, Chemicon MAB3584, 1:100), anti-HP1β (Chemicon MAB3448, 1:500), anti-HP1γ (Chemicon MAB3450, 1:500), ANA-C (Sigma ANA-C, detecting CENP-A, 1:15), anti-NDR1/2 (Millipore MABS56, 1:500) Anti-NDR-N-terminal (gift from Brian A Hemmings), anti-GFP (Covance 118R, 1:500), anti-HA, anti-FLAG (M2 FLAG Sigma F3165, 1:500), anti-Mad1 (Sigma M8069, 1:100) and anti-α-tubulin (Sigma T5168, WB-1:5,000, IF- 1:2,000), γ-tubulin (Sigma, T5792, 1:2,000), H3K9-me [3] (Upstate 07-523, 1:500) anti-phospho H3Ser 10 (Upstate 06-570, 1:600), anti-geminin (Santa Cruz sc13015, 1:300) and anti-Sgo1 (gift from Hongtao Yu). Uncropped scans of the WBs are provided in Supplementary Fig. 6 . Generation of phospho-specific HP1α.antibody Abgent custom services were used to generate and purify the phospho-specific antibody against the modified peptide SNKRKSNFBNSADDIKSKKKRC. The antibodies are purified using peptide affinity purification by Abgent custom services. The peptides are conjugated to solid phase packed in columns for purification purposes. Filtered sera are passed through non-phospho peptide (SNKRKSNFSNSADDIKSKKKRC) column and bound antibody is eluted. The pass through is then loaded to phosho-peptide column. Bound antibody is eluted as the phospho-antibody. Cell synchronization U2OS cells were synchronized at different stages of the cell cycle either by double thymidine block and release or nocodazole block and release. In brief, cells were grown in the presence of 2 mM thymidine for 24 h. After the first block, thymidine was removed by repeatedly washing the cells in PBS and cells were released for 12 h in fresh medium. Finally, cells were synchronized at G1/S by further growing them in the presence of 2 mM thymidine for 24 h. The cells were released in fresh medium for 4 h to collect them in S phase; 8 h for G2 phase and monitored for appearance of rounded cells for mitosis. Alternately, cells were synchronized at prometaphase by treating them with 50 ng ml −1 nocodazole for 12–16 h. G1 population was collected by washing the nocodazole-arrested cells in PBS and releasing them in the fresh medium for 5–6 h. Synchronized samples were evaluated by flow cytometry and immunoblot analysis. Immunoprecipitation and flow cytometry For co-IP, T7/HA-tagged WT and various mutants of NDR1 were co-transfected with YFP-tagged HP1α (both WT and mutants) in U2OS cells. Cells were lysed, 24 h post-transfection, in IP buffer (50 mM HEPES (pH 7.9), 5% glycerol, 200 mM KCl, 0.1% Triton X and 1 mM CaCl2 supplemented with protease and phosphatase inhibitors and 0.5 μM okadaic acid) followed by treatment with 2 U of micrococcal nuclease (Sigma) for 20 min at room temperature. Digestion was stopped by the addition of 0.5 M EDTA. After pre-clearing with Gammabind Sepharose beads for 1 h, the lysates were incubated with appropriate antibody-conjugated agarose overnight. The beads were washed in the same IP buffer and finally denatured by the addition of Laemmli buffer. The complex was analysed by WB. Uncropped WBs have been supplied in Supplementary Fig. 6 . For flow cytometry, cells were fixed in chilled ethanol overnight after resuspending in PBS+1% NGS. After two rounds of washing, cells were resuspended in PBS+1% NGS with 120 μg ml −1 propidium iodide and 10 μg ml −1 RNase A followed by 30 min incubation at 37 °C. DNA content was measured by flow cytometry. Immunofluorescence analysis The 2-6-3 CLTon and U2OS/HeLa cells were either fixed in ice-cold methanol at −20 °C or 2% paraformaldehyde for 15 min at room temperature. The cells were permeabilized in 0.5% Triton X-100 in PBS for 7 min, stained with 4′,6-diamidino-2-phenylindole (DAPI) followed by washing in PBS and finally were mounted in either p -phenylenediamine (PPD) or Vectashield (Vector Laboratories Inc.). For Ser 95-specific phospho-antibody, cells were first pre-extracted in 0.3% CSK buffer for 3 min followed by 2% paraformaldehyde fixation for 15 min. Antibody staining was carried out using standard procedures. A Zeiss Axioimager z1 fluorescence microscope (Carl Zeiss Inc.) equipped with Chroma filters (Chroma Technology) was used for cellular examination. Axiovision software (Carl Zeiss) was used to collect digital images from a Hamamatsu cooled charge-coupled device camera. Images were also acquired using a Delta Vision optical sectioning deconvolution instrument (Applied Precision) on an Olympus microscope. For Fig. 4 (and Supplementary Fig. 3 ), images were acquired using a deltavision optical sectioning microscope. For individual images, six sections of 0.3 μm were used for processing by deconvolution and quick projection. Depletion of human NDR1/2 Two siRNAs targeting human NDR1 (IDT, USA) against 3′-UTR (sense: 5′-CCAAUAUGUCAUAGUAAAGUCUCCT-3′, anti-sense: 3′-GUGGUUAUACAGUAUCAUUUCAGAGGA-5′) and cds (sense: 5′-AGAAAUAGACGUCAGCUAGCCUUCT-3′, anti-sense: 3′-UUUCUUUAUCUGCAGUCGAUCGGAAGA-5′) were delivered into cells twice at a gap of 24 h, at a final concentration of 10 μM, mediated by Lipofectamine RNAimax (Invitrogen). siRNA against HP1α and control luciferase have been described elsewhere [70] . Sequence of siRNA targeting human HP1α against 3′-UTR are as follows: sense: 5′–GACAUGUUGAGAUGGAAAGGAUGTT-3′, anti-sense: 3′-GACUGUACAACUCUACCUUUCCUACAA-5′. pTER-NDR1/2 constructs were used to express tetracyclin inducible shRNA against NDR1 and 2 to allow stable inducible knockdown of targeted proteins (a kind gift from Dr B Hemmings) [46] . Doxycycline (2 μg ml −1 ) was added to induce the shRNA expression for 5 days, followed by lysis and immunoblot analysis. shRNA against firefly luciferase was used as a control for these studies. Kinase assay and phos tag analysis In vitro kinase assay was performed either using GST-tagged human NDR1 purified from baculovirus-infected Sf9 cells (Sigma) or from HEK293 cells that were transfected with HA-tagged version of NDR kinase as described [40] with minor modifications. In brief, HEK293 cells were transfected with HA-NDR1 WT and were stimulated with 1μM okadaic acid (Sigma) for 1 h. The kinase was immunoprecipitated using anti-HA agarose from transfected HEK293. The HA-NDR1 was eluted by peptide elution. In vitro kinase assays was performed by incubating purified GST-tagged HP1α, its truncated mutants and GST-tagged/the eluted kinase for 30 min at 30 °C in the presence of [γ-32P] ATP in kinase buffer (25 mM Tris pH 7.5, 10 mM MgCl 2 ,100 μM ATP, 1 mM dithiothreitol). The reaction was stopped by boiling the samples in Laemmli buffer for 5 min at 95 °C. Samples were resolved on SDS–PAGE, stained with Coomassie blue and exposed to a phosphorimager (Amersham Biosciences). To detect the phosphorylation based on band shift, phos-Tag SDS–PAGE was employed according to the manufacturer’s protocol (AAL-107; NARD Institute, Amagasaki, Japan). Protein samples treated with CIP (NEB, USA) was used as a dephosphorylated control. How to cite this article: Chakraborty, A. et al. Dynamic phosphorylation of HP1α regulates mitotic progression in human cells. Nat. Commun. 5:3445 doi: 10.1038/ncomms4445 (2014).